Tracking axonal action potential propagation on a high-density microelectrode array across hundreds of sites Axons are traditionally considered stable transmission cables, but evidence of the regulation of action potential propagation demonstrates that axons may have more important roles. However, their small diameters render intracellular recordings challenging, and low-magnitude extracellular signals are difficult to detect and assign. Better experimental access to axonal function would help to advance this field. Here we report methods to electrically visualize action potential propagation and network topology in cortical neurons grown over custom arrays, which contain 11,011 microelectrodes and are fabricated using complementary metal oxide semiconductor technology. Any neuron lying on the array can be recorded at high spatio-temporal resolution, and simultaneously precisely stimulated with little artifact. We find substantial velocity differences occurring locally within single axons, suggesting that the temporal control of a neuron’s output may contribute to neuronal information processing. Evidence has shown that neocortical axons may have more important roles in neural computation than generally considered, namely, by regulating action potential propagation. For example, in the cortex and hippocampus, action potentials were found to not only encode information digitally, but also in an analogue manner: graded magnitudes of action potentials encoded a neuron’s background synaptic activity by modulating neurotransmitter release [1] , [2] . Moreover, local activity of glia broadened action potential waveforms by the activation of axonal ionotropic glutamate receptors, which facilitated synaptic transmission in a specific branch [3] . In addition, activity-dependent plasticity of the timing of action potential propagation occurred on fast time scales in cortical cultures [4] . The latter may provide neurons with a means to tune temporal coding schemes, which are theoretically used by the brain to process information [5] . A number of mechanisms that could influence axonal conduction have been reported including variation in ion channel densities and kinetics [6] ; the geometry [7] of varicosities and branch points introducing delays or selectively blocking conduction [8] ; extracellular accumulation of neurotransmitters or ions [9] ; the presence and movement of mitochondria or other subcellular units affecting axial resistance [10] ; modulation via synaptic receptors receiving input from other axons [11] or glia [3] ; coupling through gap junctions or ephaptic interactions [12] ; and, for myelinated axons, variation in myelin thickness [13] or spacing of nodes of Ranvier. For reviews on axonal information processing, see refs 14 , 15 , 16 , 17 . However, collecting physiological data from axons has been challenging owing to the small diameter of neocortical axons (0.08–0.4 μm) [15] . In particular, methods to spatially track the propagation of their action potentials at more than two sites are lacking. For many decades, the only method available for accessing axonal function involved evoking antidromic (propagation towards the soma) action potentials in axons by extracellular stimulation at a specific site of the axon and then recording elicited somatic responses [18] , [19] . Whole-cell patch recording of a relatively large 3–6 μm diameter axonal bleb [1] , bouton [2] , or the Calyx of Held [20] or, alternatively, cell-attached patch recordings of a smaller diameter axonal structure (down to ~1 μm) [17] offer techniques to measure orthodromic action potentials (propagation away from the soma). Moving beyond two sites, silicon nanowire transistors extracellularly tracked propagation at tens of sites. However, this neuron was isolated with its axon constrained to grow along a one-dimensional line [21] , and the evidence is debated [22] . To allow for detection at a few sites using commercial microelectrode arrays (MEA), small extracellular axonal signals can be amplified by confining growth within polydimethylsiloxane microtunnels [23] . Instead of using electrophysiological methods, fluorescent molecules sensitive to voltage [24] , Ca 2+ (ref. 25 ) or Na + (ref. 26 ) can serve to optically detect axonal signals. For example, improved voltage-sensitive dye techniques imaged action potentials travelling in Purkinje cell axon collaterals, although cells remained viable for only a few seconds of total illumination [27] . However, optical techniques subject cells to phototoxicity and photobleaching within seconds to hours. Furthermore, optical reporter molecules interfere with cell physiology, such as cellular calcium buffers or membrane capacitance, to the point of affecting action potential conduction [24] . New tools providing sufficient spatio-temporal resolution and signal quality to detect signals from submicron diameter axons would help to advance this field. Our objective was to provide high spatio-temporal resolution experimental access to track the propagation of action potentials. The present paper reports on methods to non-invasively detect, assign and track the pathways of stimulation-triggered axonal signals across hundreds of electrodes. Dendritic signals can also be detected after somatic depolarization. Our data experimentally show, to our knowledge for the first time, that many-fold velocity differences exist locally within a single neocortical axon. Furthermore, tracking of a single axon over several days demonstrates that the velocity profile varied significantly across days. The power of the methods is best demonstrated viewing the Supplementary Movies . To visualize the action potential propagation, primary dissociated co-cultures of cortical neurons and glia were grown over a custom MEA that is based on complementary metal oxide semiconductor (CMOS) technology. The array contains 11,011 electrodes within a 2.0 × 1.8-mm 2 area that are packed densely enough to touch any neuron lying on the array [28] . Electrodes exhibit signal-to-noise ratios up to 180σ noise for somatic signals and often between 1 and 2σ noise for axonal signals. Importantly, each electrode can be used to issue spatially precise and confined stimuli that produce low artifact. Axons were spatially unconstrained and embedded among other neurons, allowing the possibility to investigate their computational roles within cultured neuronal networks in future studies. CMOS-based MEAs allow precise recording and stimulation Cortical networks were grown over 11,011-electrode, CMOS-based MEAs [28] . The devices provide the ability to simultaneously stimulate and record from any neuron lying on the array surface, non-invasively and for durations of months. To ensure excellent signal quality (low noise) at the given high electrode density (17.8 μm pitch; 8.2 × 5.8 μm 2 area per electrode), a matrix of switches was embedded in the device to simultaneously connect arbitrary subsets of electrodes to 126 on-chip read-out channels placed at the periphery of the array. The electrode configurations could be changed or re-routed within milliseconds. 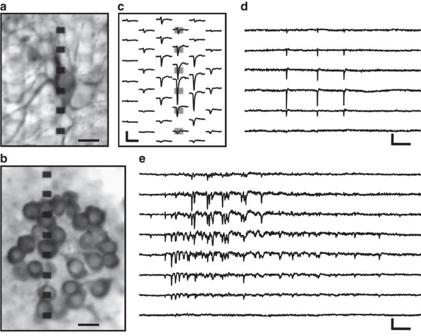Figure 1: Immunofluorescent images of neurons grown over the array and their spontaneous electrical signals. (a) Fluorescence image of an isolated neuron’s soma and dendrites stained with MAP2. Black rectangles highlight one column of electrodes located underneath the neuron and are plotted to scale (8.2 × 5.8 μm2per electrode). Scale bar, 20 μm. (b) Fluorescence image of a cluster of neurons and one highlighted column of electrodes (black rectangles). Scale bar, 20 μm. (c) Spatial distribution of action potential waveforms for the neuron ina, termed a footprint. Ten peak-aligned spikes were averaged for electrodes from all columns. The highlighted column shown inais plotted in grey inc. Scale bars, 2 ms horizontal and 200 μV vertical. (d,e) Voltage traces recorded on the electrodes marked by rectangles inaandb, respectively, during a network burst. The isolated neuron produced clear individual spikes detected on multiple electrodes (d), whereas the cluster of neurons produced overlapping spikes (e). Shrinkage during the cell fixation process or cell movement before fixation may cause some misalignment between the recorded activity and cell locations. Scale bars, 10 ms horizontal and 400 μV vertical. Figure 1 provides fluorescent images of an isolated neuron ( Fig. 1a ), a cluster of neurons ( Fig. 1b ) and their corresponding activity ( Fig. 1c–e ; Supplementary Fig. S1 , and Supplementary Movie 1 ). The isolated cell is easily identified and localized owing to its clean spikes and the spatial distribution of action potential waveforms across neighbouring electrodes, termed a footprint. The footprint in the figure exceeded a common 5σ noise spike-detection threshold at 18 electrodes. During a network burst, this neuron fired three times in its own individual burst sequence. On the other hand, the cluster of neurons fired overlapping action potentials, which makes isolating single-unit neuronal activity difficult. Similarly, we found that many axons were also simultaneously activated during network bursting, which makes the propagation of spontaneous action potentials difficult to discern and track. Algorithms are being developed to assign signals to their respective neurons, commonly termed spike-sorting, by comparing signal waveforms across neighbouring electrodes [29] , [30] . Alternatively, such difficulties can be minimized by analysing responses to electrical stimulation, as discussed in the next sections. Figure 1: Immunofluorescent images of neurons grown over the array and their spontaneous electrical signals. ( a ) Fluorescence image of an isolated neuron’s soma and dendrites stained with MAP2. Black rectangles highlight one column of electrodes located underneath the neuron and are plotted to scale (8.2 × 5.8 μm 2 per electrode). Scale bar, 20 μm. ( b ) Fluorescence image of a cluster of neurons and one highlighted column of electrodes (black rectangles). Scale bar, 20 μm. ( c ) Spatial distribution of action potential waveforms for the neuron in a , termed a footprint. Ten peak-aligned spikes were averaged for electrodes from all columns. The highlighted column shown in a is plotted in grey in c . Scale bars, 2 ms horizontal and 200 μV vertical. ( d , e ) Voltage traces recorded on the electrodes marked by rectangles in a and b , respectively, during a network burst. The isolated neuron produced clear individual spikes detected on multiple electrodes ( d ), whereas the cluster of neurons produced overlapping spikes ( e ). Shrinkage during the cell fixation process or cell movement before fixation may cause some misalignment between the recorded activity and cell locations. Scale bars, 10 ms horizontal and 400 μV vertical. Full size image Extracellular stimulation directly activated neural tissue with low artifact ( Fig. 2 ) and high spatial precision ( Fig. 3 ). Low artifact is necessary in order to observe the signals produced by activated neurons. High spatial precision reduces the problem of signal overlap by reducing the number of activated neurons. Stimulation artifacts affected all electrodes while applied, but only voltage traces for electrodes located within an ~100-μm radius of the stimulation site were saturated ( Fig. 2a ). Traces from ~99% of electrodes are within the measurement range after the cessation of the stimulus pulse so that much of the evoked activity is available for analysis. 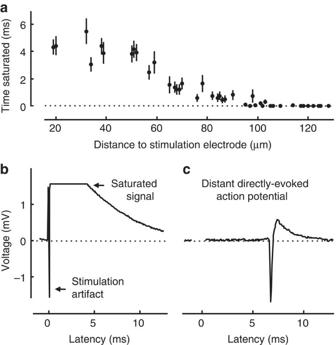Figure 2: Biphasic voltage stimulation saturated signals only on nearby recording electrodes. (a) The duration of a saturated signal occurring after stimuli is plotted versus distance from the stimulation electrode (mean±s.e.m.;N=18 stimulation electrodes from five CMOS-based MEAs). Stimuli consisted of biphasic voltage pulses between 100 and 200 μs duration per phase and between ±400 and 800 mV amplitude. On an average, signals on <1% of the electrodes become saturated after a stimulus. (b) A raw voltage trace recorded at an electrode neighbouring a stimulation electrode saturated for about 4 ms (flat line). The stimulus was applied at time zero. (c) A raw voltage trace recorded at an electrode located 1.46 mm away from a stimulation electrode did not saturate; the signal during stimulation was blanked in software before recording. Synaptic activity was pharmacologically blocked (seeMethods), demonstrating that the stimulus directly evoked an action potential that antidromically propagated until evoking the exceptionally large somatic action potential plotted here. Figure 2: Biphasic voltage stimulation saturated signals only on nearby recording electrodes. ( a ) The duration of a saturated signal occurring after stimuli is plotted versus distance from the stimulation electrode (mean±s.e.m. ; N =18 stimulation electrodes from five CMOS-based MEAs). Stimuli consisted of biphasic voltage pulses between 100 and 200 μs duration per phase and between ±400 and 800 mV amplitude. On an average, signals on <1% of the electrodes become saturated after a stimulus. ( b ) A raw voltage trace recorded at an electrode neighbouring a stimulation electrode saturated for about 4 ms (flat line). The stimulus was applied at time zero. ( c ) A raw voltage trace recorded at an electrode located 1.46 mm away from a stimulation electrode did not saturate; the signal during stimulation was blanked in software before recording. Synaptic activity was pharmacologically blocked (see Methods ), demonstrating that the stimulus directly evoked an action potential that antidromically propagated until evoking the exceptionally large somatic action potential plotted here. 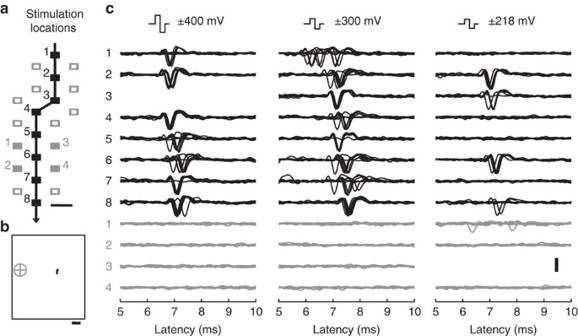Figure 3: Stimuli activated neural tissue with high spatial precision. (a) Locations of stimulation electrodes that directly evoked (black boxes) or did not evoke (empty or filled grey boxes) action potentials detected at a soma located ~890 μm away. Electrodes are plotted to scale 8.2 × 5.8 μm2, and the electrode numbering and line arrow indicate the orthodromic propagation direction. Scale bar, 20 μm. (b) Location of the soma (grey crosshair) with respect to the stimulation electrodes (black line) and the geometry of the array (box). Scale bar, 200 μm. (c) Voltage traces of somatic action potentials elicited by biphasic voltage stimuli. Traces in response to eight stimuli are overlaid for each of three stimulation magnitudes (indicated at the top), plotted for all effective (black) and four ineffective stimulation sites (grey at the bottom). Stimulation electrode locations are represented as numbered boxes ina. Towards the end of the experiment, the algorithm that randomly sets electrode configurations took progressively longer to route the remaining electrodes. Therefore, owing to time considerations, not all electrodes were selected (that is, black electrode 3 in the first column and grey electrode 3 in the last column). Scale bar, 200 μV. Full size image Figure 3: Stimuli activated neural tissue with high spatial precision. ( a ) Locations of stimulation electrodes that directly evoked (black boxes) or did not evoke (empty or filled grey boxes) action potentials detected at a soma located ~890 μm away. Electrodes are plotted to scale 8.2 × 5.8 μm 2 , and the electrode numbering and line arrow indicate the orthodromic propagation direction. Scale bar, 20 μm. ( b ) Location of the soma (grey crosshair) with respect to the stimulation electrodes (black line) and the geometry of the array (box). Scale bar, 200 μm. ( c ) Voltage traces of somatic action potentials elicited by biphasic voltage stimuli. Traces in response to eight stimuli are overlaid for each of three stimulation magnitudes (indicated at the top), plotted for all effective (black) and four ineffective stimulation sites (grey at the bottom). Stimulation electrode locations are represented as numbered boxes in a . Towards the end of the experiment, the algorithm that randomly sets electrode configurations took progressively longer to route the remaining electrodes. Therefore, owing to time considerations, not all electrodes were selected (that is, black electrode 3 in the first column and grey electrode 3 in the last column). Scale bar, 200 μV. Full size image Often, an action potential was evoked in an axon and propagated antidromically (and orthodromically) up to tens of milliseconds [4] , [31] until it depolarized its soma at a distant site ( Fig. 2c ; directly visible in Figs 4a and 8d–e and Supplementary Movies 1,2 and indirectly demonstrated previously [4] , [32] , [33] ). Such directly evoked somatic spikes can be identified by a high reliability of occurrence, low temporal jitter and consistent waveform. The directly evoked nature has been verified as they still occurred when synaptic activity was blocked ( Figs 2c and 4a ). The spike in Fig. 2c had the largest magnitude we recorded: −1.7 mV 0-peak or 180 σ noise , with a jitter in latency of 50 μs rms over 30 trials. (Lower-spike heights are often seen such as those in Fig. 1 ). For comparison, spike-detection algorithms commonly consider spikes exceeding 5σ noise to represent valid action potentials. 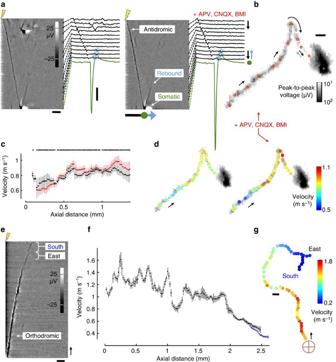Figure 4: Antidromic and orthodromic action potentials and velocities. (a) Mean voltages calculated from 60 stimulation trials along a pathway for a neuron bathed in standard media (left) and media supplemented by the synaptic receptor antagonists 2-amino-5-phosphonovaleric acid (APV), CNQX and bicuculline methiodide (BMI; right; seeMethods). Heat maps from 95 electrodes and a subset of their averaged raw traces plotted next to the heat maps show a propagating antidromic action potential, subsequent somatic depolarization (green) and an action potential rebounding from the soma (highlighted in blue). Arrows indicate the propagation direction and yellow bolts indicate the stimulation time. Scale bars, 1 ms horizontal; 100 μV vertical. (b) A footprint of the pathway stitched together from 17 adjacent recording configurations represented by the peak-to-peak median voltage at each electrode (grey scale pixels). Red circles denote locations of the subset of traces ina, with synaptic antagonists. Scale bar, 100 μm. (c) Velocities froma–cwithout (black) and with (red) synaptic antagonists calculated by using a bootstrapping procedure (mean±s.d.;N=1000 bootstrap estimates from re-sampling with replacement; dots above the plot indicate significant differences,P-value <10−3, Mann–WhitneyU-test). (d) Velocity profiles (colour) along the propagation pathway without (left) and with (right) synaptic antagonists. (e–g) The same analysis was performed for an orthodromic action potential recorded in a single-electrode configuration. Propagation continued into two branches (‘East’ and ‘South’). The red cross ingindicates the stimulation electrode located near the soma, and arrows indicate the propagation direction. Scale bars, 1 ms ineand 100 μm ing. See alsoSupplementary Movie 2. Figure 4: Antidromic and orthodromic action potentials and velocities. ( a ) Mean voltages calculated from 60 stimulation trials along a pathway for a neuron bathed in standard media (left) and media supplemented by the synaptic receptor antagonists 2-amino-5-phosphonovaleric acid (APV), CNQX and bicuculline methiodide (BMI; right; see Methods ). Heat maps from 95 electrodes and a subset of their averaged raw traces plotted next to the heat maps show a propagating antidromic action potential, subsequent somatic depolarization (green) and an action potential rebounding from the soma (highlighted in blue). Arrows indicate the propagation direction and yellow bolts indicate the stimulation time. Scale bars, 1 ms horizontal; 100 μV vertical. ( b ) A footprint of the pathway stitched together from 17 adjacent recording configurations represented by the peak-to-peak median voltage at each electrode (grey scale pixels). Red circles denote locations of the subset of traces in a , with synaptic antagonists. Scale bar, 100 μm. ( c ) Velocities from a – c without (black) and with (red) synaptic antagonists calculated by using a bootstrapping procedure (mean±s.d. ; N =1000 bootstrap estimates from re-sampling with replacement; dots above the plot indicate significant differences, P- value <10 −3 , Mann–Whitney U -test). ( d ) Velocity profiles (colour) along the propagation pathway without (left) and with (right) synaptic antagonists. ( e – g ) The same analysis was performed for an orthodromic action potential recorded in a single-electrode configuration. Propagation continued into two branches (‘East’ and ‘South’). The red cross in g indicates the stimulation electrode located near the soma, and arrows indicate the propagation direction. Scale bars, 1 ms in e and 100 μm in g . See also Supplementary Movie 2 . Full size image Stimulation activated only neurons local to a given electrode. This is shown in Fig. 3 , where a group of electrodes neighbouring a putative axon were stimulated while monitoring the antidromic responses at its distant soma. The four ineffective sites, marked and numbered in grey, completely surrounded an effective site (site 6). This indicates that the effective spatial extent of the stimuli beyond the electrode area is less than the maximum edge-to-edge electrode spacing of 13 μm. Decreasing stimulation magnitude from ±400 mV to ±218 mV further increased precision, as judged by previously effective sites that no longer elicited a response. Precision will depend on electrode conditions and the local environment, such as the relative position of electrodes with respect to axons and cells, as well as on the presence of experimental devices affecting the elicited electric field [23] . Stimuli-triggered averaging of propagating action potentials In addition to somatic action potentials, smaller signals propagating through axons and dendrites were observed by calculating the mean or median voltage traces in response to stimulation ( Figs 4 , 5 , 6 and 8d and Supplementary Movies 1–3 ). Stimulation-triggered electrical images and movies were compiled by scanning ~100 recording configurations across the whole 1.8 × 2.0 mm 2 array, whereas stimuli were applied at a single electrode multiple times per configuration. Although recorded at different time points, the stitched-together configurations were compatible because voltage stimulation evoked action potentials reliably with high precision, time-locked to the downswing of the biphasic stimulation pulse [4] . Afterwards, electrodes along a pathway were grouped together in a single configuration to provide fast tracking of signal propagation in a specific axon ( Fig. 4e–g ). 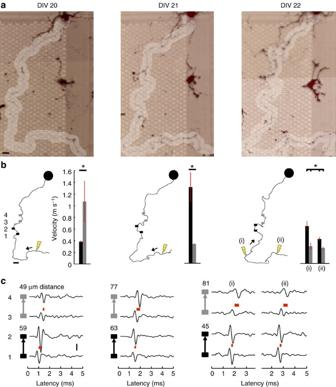Figure 5: Velocity differences existed between neighbouring segments. (a) Live-cell images of a neuron expressing red fluorescent protein (RFP) were taken between DIV 20 and DIV 22. The axonal trunk is highlighted for clarity. Images are a montage of two frames. Scale bar, 40 μm. (b) Stimuli were repeatedly applied to a single electrode (stimulation location indicated by the yellow bolt) over 3 days (repeated once on DIV 22 at a different site a few minutes later; see (i) and (ii)), whereas a series of eight recording configurations were scanned across the axon. Velocities were measured at two isolated sections of the axon (mean±s.d.;N=1,000 bootstrap estimates from re-sampling with replacement; asterisks denote significant differences, andP-value <10−3for every combination, Mann–WhitneyU-test). The recording electrodes are marked by black and grey rectangles, and the antidromic propagation direction is shown by arrows. Scale bar, 40 μm. (c) Mean voltages from 90 stimulation trials were used to calculate the relative action potential timing (red bars) at the recording electrodes numbered inb. Stimulation artifact was removed by subtracting a curve fit to the signal (Supplementary Fig. S4). Scale bar, 5 μV. See alsoSupplementary Movie 3. Figure 5: Velocity differences existed between neighbouring segments. ( a ) Live-cell images of a neuron expressing red fluorescent protein (RFP) were taken between DIV 20 and DIV 22. The axonal trunk is highlighted for clarity. Images are a montage of two frames. Scale bar, 40 μm. ( b ) Stimuli were repeatedly applied to a single electrode (stimulation location indicated by the yellow bolt) over 3 days (repeated once on DIV 22 at a different site a few minutes later; see (i) and (ii)), whereas a series of eight recording configurations were scanned across the axon. Velocities were measured at two isolated sections of the axon (mean±s.d. ; N =1,000 bootstrap estimates from re-sampling with replacement; asterisks denote significant differences, and P- value <10 −3 for every combination, Mann–Whitney U -test). The recording electrodes are marked by black and grey rectangles, and the antidromic propagation direction is shown by arrows. Scale bar, 40 μm. ( c ) Mean voltages from 90 stimulation trials were used to calculate the relative action potential timing (red bars) at the recording electrodes numbered in b . Stimulation artifact was removed by subtracting a curve fit to the signal ( Supplementary Fig. S4 ). Scale bar, 5 μV. See also Supplementary Movie 3 . 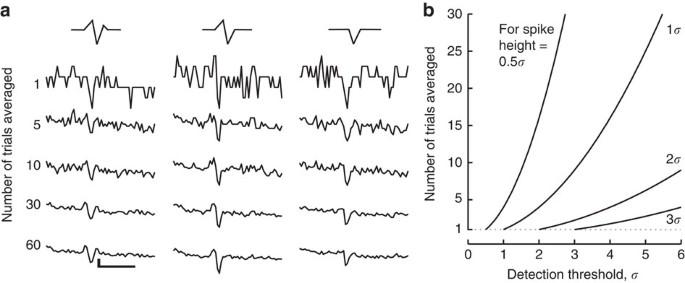Figure 6: Extracellular detection of propagating action potentials and the effect of averaging. (a) Examples of elicited tri-, bi- and mono-phasic spikes detected at three sites (columns) along the same axon. The top row shows individual raw traces, and the other rows show traces averaged as indicated. Scale bars, 1 ms horizontal, 10 μV vertical. (b) The amount of averaging necessary to detect a spike with a given height (0.5–3σ) with respect to the detection threshold; note that 5σnoiseis a common threshold to reliably detect somatic spikes. The number of trials necessary to average is equal to the square of the detection threshold divided by the spike height:N=(T/H)2. Full size image Figure 6: Extracellular detection of propagating action potentials and the effect of averaging. ( a ) Examples of elicited tri-, bi- and mono-phasic spikes detected at three sites (columns) along the same axon. The top row shows individual raw traces, and the other rows show traces averaged as indicated. Scale bars, 1 ms horizontal, 10 μV vertical. ( b ) The amount of averaging necessary to detect a spike with a given height (0.5–3σ) with respect to the detection threshold; note that 5σ noise is a common threshold to reliably detect somatic spikes. The number of trials necessary to average is equal to the square of the detection threshold divided by the spike height: N =( T / H ) [2] . Full size image The velocities measured from axonal spikes ( Fig. 4a ) were different at different locations along a pathway for both antidromic ( Fig. 4c ) and orthodromic ( Fig. 4f ) propagation. Interestingly, an action potential rebounding from the soma was tracked until a bend in the pathway in Fig. 4b . The rebound could have followed a different colocalized neurite, or alternatively the same neurite if generated by an impedance mismatch at the soma [15] , [34] . Local differences in velocity also occurred when synaptic activity was blocked ( Fig. 4c ). Although the presence of network activity seems to influence relative differences in velocities between the two conditions in Fig. 4c , any conclusions about the underlying mechanisms cannot be drawn yet. In Fig. 4f , the velocities measured from axonal spikes ( Fig. 4e ) were up to fivefold slower at the putatively thinner distal branches ( Fig. 4g ‘East’ and ‘South’; P -value <10 −6 , Mann–Whitney U -test), a trend theoretically supported by velocity being inversely proportional to fibre diameter [34] . Data in Fig. 4a–d were acquired by scanning a series of 108 rectangular recording configurations across the whole array, with 60 stimuli (4 Hz) sent per configuration. For Fig. 4e , a soma was initially identified by its antidromic activation as in Fig. 4a . To then produce orthodromic action potentials, the protocol was repeated but with stimulation instead applied at the electrode that had recorded the largest somatic voltage peak for the respective neuron (see Fig. 1c ). Finally, electrodes under the activated axon were gathered into a single configuration and 60 stimuli (4 Hz) were applied to produce the data here. Velocity differences existed spatially between neighbouring segments, temporally between days and functionally between sites of initiation. In Fig. 5 and Supplementary Movie 3 , recordings were correlated to live-cell fluorescence images, and velocities were tracked over 3 days. Two continuous and isolated sections of the axon were optically identified to ensure that recorded signals were from the same axon and that axial distance could be measured reliably. Significant differences in velocity between neighbouring axonal segments, across days, and with respect to different stimulation sites, were observed ( P- value <10 −6 for every combination, Mann–Whitney U -test). At day in vitro (DIV) 21, velocity differed fourfold compared with its neighbouring segment and to the previous day. To verify that differences were robust to errors in measuring distance, we hypothetically increased the measured distance between one pair of electrodes (electrodes 3 and 4), while holding the distance between the other pair constant (electrodes 1 and 2), for the smallest (DIV 22 (ii) ) and largest (DIV 21) differences observed. Distances would need to be in error by unrealistic values of 51 μm (62%) and 221 μm (387%), respectively, before velocities were no longer significantly different. For each of the four experiments, data were stitched together from a series of six recording configurations, with 90 stimuli (2.5 Hz) applied per configuration. Lipofection was used to sparsely transfect neurons with a plasmid expressing a red fluorescent protein (DsRedExpress [35] ) at DIV 17. For data not accompanied by images, velocities were calculated from linear regressions of axial distance versus spike latency of sites along the axon using 300 μm-sized axial windows stepped by 17.8 μm, the electrode pitch (all R 2 >0.9). The measured velocities ( Figs 4c, f , 5b , 7d and ) suggest that propagation occurred in unmyelinated fibres [8] , [14] , [16] , [21] . Velocities were calculated assuming straight paths between recording electrodes, whereas the actual path may curve. To estimate the error introduced by this assumption, the amount of curvature was quantified from live-cell images of seven putative axons and incorporated into the distribution of distances used during bootstrapping ( Supplementary Fig. S2 ). Bootstrapping (re-sampling with replacement 1000 times) was used to estimate the accuracy of our velocity measurements and to allow for statistical testing of velocity comparisons. Although dendritic signals occurring after somatic depolarization could be recorded, we do not have any evidence that action potentials could be elicited by dendritic stimulation (see next sub-section and also Discussion). Therefore, in order to ensure that velocity measurements characterized axonal signals and did not include dendritic spikes, we only analysed propagation pathways identified between a successfully tested stimulation site and subsequently evoked soma. For simplicity, spike timing was determined according to the occurrence of the negative extracellular peak. Consistent results were obtained when alternatively considering the occurrence of the positive peak, the point of maximum slope between the peaks, and by the peak of the signal convolved by a stereotypical axonal spike waveform. 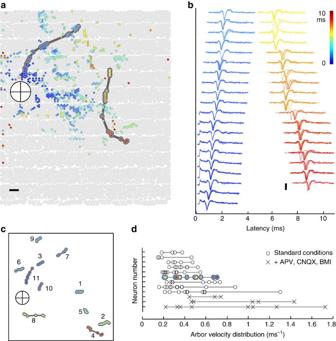Figure 7: Spatio-temporal reconstruction of segments of a neuronal arbour. (a) Stimulated electrodes are plotted that evoked (coloured by median latency until detection of somatic action potentials) or did not evoke (light grey) somatic action potentials at the crosshair (its radius indicates the approximate area affected by saturated signals after a stimulus; seeFig. 2a). Scale bar, 100 μm. (b) Somatic action potentials evoked by stimuli applied to different electrodes (rows) along two putative arbour pathways (dark grey in (a)). Colour again represents latency but also maps electrodes to their positions ina. Scale bar, 200 μV. (c) Locations of arbour sections of the neuron inaused to calculate velocities in the colour-matched circles ind, numbered by increasing velocity. (d) Propagation velocities estimated by a linear regression of distance versus latency from 89 arbour sections (circles in standard conditions; crosses when synaptic activity was blocked) from 12 neurons (horizontal lines, colour matches (a–c);R2values were 0.93 mean±0.08 s.d.;N=89). See alsoSupplementary Movie 4. Figure 7: Spatio-temporal reconstruction of segments of a neuronal arbour. ( a ) Stimulated electrodes are plotted that evoked (coloured by median latency until detection of somatic action potentials) or did not evoke (light grey) somatic action potentials at the crosshair (its radius indicates the approximate area affected by saturated signals after a stimulus; see Fig. 2a ). Scale bar, 100 μm. ( b ) Somatic action potentials evoked by stimuli applied to different electrodes (rows) along two putative arbour pathways (dark grey in ( a )). Colour again represents latency but also maps electrodes to their positions in a . Scale bar, 200 μV. ( c ) Locations of arbour sections of the neuron in a used to calculate velocities in the colour-matched circles in d , numbered by increasing velocity. ( d ) Propagation velocities estimated by a linear regression of distance versus latency from 89 arbour sections (circles in standard conditions; crosses when synaptic activity was blocked) from 12 neurons (horizontal lines, colour matches ( a – c ); R 2 values were 0.93 mean±0.08 s.d. ; N =89). See also Supplementary Movie 4 . Full size image Averaging revealed extracellular spikes of propagating action potentials that were characteristically bi- or tri-phasic, with a noticeable positive-first phase. The last positive phase was occasionally absent ( Fig. 6a ). Such spikes were often observed between 1 and 2σ noise . For an averaged trace to exceed a 5σ noise detection threshold, 7–25 trials would be necessary: N =(detection threshold/spike height) [2] ( Fig. 6b ). Using this threshold on the footprint in Fig. 4b ( N =60 trials averaged), ~200 electrodes detected the propagating action potential (soma excluded). To generate the footprint, peak-to-peak median voltages were calculated for electrodes neighbouring the propagation axis, as found within a 60-μm or three-electrode radius around the time of the passing spike (negative peaks within ±1 sample, equal to ±50 μs, of each other). For clarity in the figure, electrodes not in configurations (~3%) were assigned the average value of their adjacent electrodes; a non-adjusted plot is given in Supplementary Fig. S3 for comparison. The axon footprint had a non-uniform signal height along its axis, which sometimes became very small. This could be due a number of factors including the relative location with respect to the electrodes or, for example, if an axon climbed over other cells; the presence of other neurons and glia affecting spreading or sealing resistances; or variations in available ion channels. In contrast to axonal-propagating action potentials, extracellular somatic spikes had an initial predominant negative phase followed by a positive rebound of varying magnitude ( Figs 2c , 3c and 4a ). This was caused in part by the soma acting as a source for later depolarizing components [36] . Actual somatic spike shapes will also depend on the factors listed above. Distributed stimuli to create a spatio-temporal neuronal map By taking advantage of the property that a directly evoked action potential can propagate until depolarizing its soma at a distant electrode, a neuronal arbour was partially reconstructed spatially and temporally by scanning stimuli across the array while recording responses from one soma ( Figs 7 and 8b and Supplementary Movie 4 ). By then plotting the locations of stimulation electrodes that successfully evoked somatic action potentials, continuous lengths and some branching of a neuron’s arbour were partially reconstructed at 638 locations ( Fig. 7a ). To avoid inclusion of falsely identified segments that would occur as a consequence of coincidental spontaneous spikes, a location was only accepted if at least half of the stimuli (applied eight times per electrode; 5 Hz) evoked an action potential at the soma within, considering jitter, a 0.5-ms time window. Figure 7b shows somatic spikes in response to stimuli applied along two putative axonal pathways. Conduction velocities, again found from the slope of a linear regression of distance versus latency, further suggest that action potential velocity varied at different locations within a neuron ( Fig. 7c–d ; maximum velocity differences per neuron averaged 3.7±2.0-fold, mean±s.d. ; N =12 neurons and 89 arbour segments). As also observed by using the previous method, variation remained when synaptic activity was blocked ( Fig. 7d ). 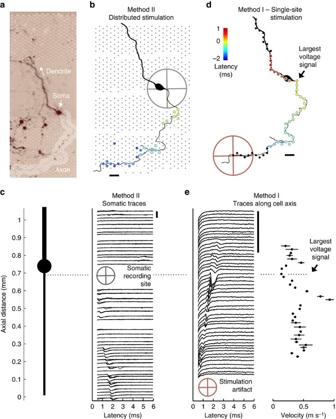Figure 8: Both methods applied to track an axon of a red fluorescent protein (RFP)-expressing neuron. (a) Live-cell image at DIV 21 of a neuron transfected with RFP at DIV 17. The axonal trunk is highlighted for clarity. The image is a montage of three frames. Scale bar, 40 μm. (b) Stimulated electrodes that evoked (coloured by median latency until action potential detection) or did not evoke (light grey) ‘somatic’ action potentials at the crosshair (its radius indicates the approximate area affected by saturated signals after a stimulus; seeFig. 2). Scale bar, 40 μm. (c) Overlaid voltage traces recorded at the soma in response to stimuli applied along the main axonal and dendritic trunks. Stimulation electrode locations are the same as the recording electrode locations indicated by dots ind. Scale bar, 400 μV. (d) Stimuli were repeatedly applied to a single electrode (red cross), whereas a series of 12 recording configurations were scanned across the neuron. Latencies (colour) with respect to the largest voltage signal (arrow) are plotted for detected action potentials. Scale bar, 40 μm. (e) Mean voltages from 90 stimulation trials recorded along the main axonal and dendritic trunks and soma. Recording electrode locations are indicated ind. Velocities were calculated by using a bootstrapping procedure (mean±s.d.;N=1,000 bootstrap estimates from re-sampling with replacement). Scale bar, 400 μV. See alsoSupplementary Movie 5. Figure 8: Both methods applied to track an axon of a red fluorescent protein (RFP)-expressing neuron. ( a ) Live-cell image at DIV 21 of a neuron transfected with RFP at DIV 17. The axonal trunk is highlighted for clarity. The image is a montage of three frames. Scale bar, 40 μm. ( b ) Stimulated electrodes that evoked (coloured by median latency until action potential detection) or did not evoke (light grey) ‘somatic’ action potentials at the crosshair (its radius indicates the approximate area affected by saturated signals after a stimulus; see Fig. 2 ). Scale bar, 40 μm. ( c ) Overlaid voltage traces recorded at the soma in response to stimuli applied along the main axonal and dendritic trunks. Stimulation electrode locations are the same as the recording electrode locations indicated by dots in d . Scale bar, 400 μV. ( d ) Stimuli were repeatedly applied to a single electrode (red cross), whereas a series of 12 recording configurations were scanned across the neuron. Latencies (colour) with respect to the largest voltage signal (arrow) are plotted for detected action potentials. Scale bar, 40 μm. ( e ) Mean voltages from 90 stimulation trials recorded along the main axonal and dendritic trunks and soma. Recording electrode locations are indicated in d . Velocities were calculated by using a bootstrapping procedure (mean±s.d. ; N =1,000 bootstrap estimates from re-sampling with replacement). Scale bar, 400 μV. See also Supplementary Movie 5 . Full size image However, the overall time needed for applying stimuli distributed to all electrodes is a limitation when estimating velocities. To gather the data ( Figs 7 and 8b ), ~77,000 stimuli were applied to over 9000 electrodes (82%) in random order over 5 h. Neuronal plasticity occurring during the 5 h could potentially alter velocity calculations. Performing only eight stimulation trials per electrode reduced the accuracy. Towards the end of the experiment, the algorithm that sets electrode configurations took progressively longer to route the remaining electrodes. Therefore, owing to time considerations, not all electrodes were selected. In contrast, the stimuli-triggered averaging method required between tens of stimuli in a few seconds for a single configuration ( Fig. 4e–g ) and up to 5700 stimuli in ~20 min to scan the whole array ( Fig. 4a–d ). The gaps in the reconstruction in Fig. 7a may have occurred due to neurites running between electrodes or climbing over other cells, variation in electrode quality or impedance necessitating different effective stimulus magnitudes, shunting from evoked inhibitory neurons and differences in local excitability. Although a distributed arbour was observed in Fig. 7 , mainly single pathways, presumably corresponding to axonal trunks, were observed by using the stimuli-triggered averaging method. This may be due to antidromic action potentials failing to orthodromically enter collaterals at branch points and/or an inability to record signals from thinner collaterals. Performing both methods together on a red fluorescent protein-expressing neuron yielded further observations ( Fig. 8 and Supplementary Movie 5 ). First, stimulation evoked a somatic response when applied along the axon, but not when applied along the dendritic trunk or in its vicinity ( Fig. 8b ). We did not find any evidence of dendritic stimulation with our electrodes probably because axons have a lower activation threshold as compared with dendrites [37] , and we were not even able to evoke all sections of an axon (that is, the incomplete arbour reconstructions in Figs 7a and 8b ). Second, dendritic signals could be recorded, and they were tracked until about 100 μm away from the soma in Fig. 8e (see also Supplementary Movie 5 ). Third, the largest magnitude ‘somatic’ spike was centred on the axon hillock and not the soma ( Fig. 8d and Supplementary Movie 5 ; also observed in four out of four additional cells and during spontaneous activity; not shown). Additional ionic current necessary to depolarize the somatic volume probably contributed to the large extracellular signal by sodium entering the cell through the high-conductance axon initial segment. In addition, significant velocity differences were observed again, and a threefold difference existed in the axon ( P -value <10 −6 , Mann–Whitney U -test). To make velocity profiles comparable to those measured in Fig. 5 , velocities were calculated between every fourth electrode (about every 60 μm). The CMOS-based MEA presented here provides a system to record and stimulate individual neocortical axons at hundreds of sites, which offers a technological advancement for the study of axonal function. Any neuron lying on the array can be detected over days and months with high spatial and temporal resolution recordings that exhibit excellent signal-to-noise. High precision stimulation that produces little artifact can be applied while recording. Two methods to detect, assign and track axonal pathways across hundreds of electrodes were presented: one based on averaging stimulus-triggered recordings and the other on spatially scanning stimuli across the array. CMOS-based MEAs hold promise to open new avenues of research but have a brief history to date. Inspired by glass-substrate-based MEAs introduced three decades ago [38] , [39] , [40] , CMOS-based MEAs have been in development during the last decade by our lab and others to interface electrogenic tissue at higher spatial resolutions [41] . For example, we previously recorded from acute cerebellar slices [42] , retinae [43] and cardiomyocytes [44] . This paper demonstrates methods for on-chip stimulation and visualization of resulting propagating action potentials. In other labs, the spread of network bursts of action potentials and functional connectivity in hippocampal cultures were analysed with a 42-μm-pitched array of 4096 electrodes [45] , [46] . Hippocampal slices or cultures and retinae have also been analysed with a 7.4-μm-pitched array of 16,384 or 32,768 open-gate field effect transistors [47] , [48] . Supporting our results, the propagation of light-evoked action potentials in retinal preparations were observed for signals averaged across ‘vectors’ of multiple trials ( N =100); one vector consisted of 3 × 3 electrodes and three time points [48] . More recently, cardiomyocytes were used to validate a 30-μm-pitched array of 16,384 stimulation electrodes that had one recording channel [49] and hippocampal cultures were used to validate a 12.2-μm-pitched array of 65,000 stimulation electrodes, without electrical recording channels, using optical detection of Ca 2+ activity [50] . Our study focused on neurites that were depolarized by extracellular electrical stimulation, which showed propagation pathways between stimulation sites and the soma. It is possible that these neurites could be either axons or dendrites, but the latter case is not expected [37] , [51] , [52] and was not observed here ( Fig. 8b ). Many studies demonstrate that the excitability of dendrites is low. For example, axonal arbours were shown to be the sites activated by extracellular stimulation when comparing chronaxies of stimulus strength-duration curves for various neuronal elements in cortical slices [37] , [51] . This is largely because of the greater abundance of voltage-sensitive sodium channels, which govern active signal propagation in axons compared with somas or dendrites. Specifically, densities were estimated between 100 and 200 channels per μm 2 for unmyelinated axons [53] and 3–10 channels per μm 2 for somas and dendrites [37] . Likewise, peak sodium current density was ~19-fold greater and activation threshold ~12 mV lower in axons than in somas in cortical slices [54] . Sodium current density per action potential in axons was three times greater than that in somas and nine times greater than that in basal dendrites, as measured by the high-speed fluorescence Na + imaging of cortical pyramidal cells [26] . Backpropagating action potentials and dendritic spikes ( Fig. 8d ) demonstrate that active propagation occurs in dendrites. However, signals strongly attenuate with distance travelled [52] . Forward propagation is attenuated at greater rates owing to arbour geometry, whereby progressively larger branch volumes require progressively greater current to continue propagation. For example, forward-propagating spikes attenuated approximately sixfold, and excitatory post-synaptic potentials 30 to 40-fold in cortical pyramidal dendrites [55] . Here we present direct measurements of substantial velocity differences occurring locally within a single neocortical axon. The measured velocities were consistent with those reported for unmyelinated axons [8] , [14] , [16] , [21] . In previous studies, velocities were regulated in a variety of species and brain structures to achieve isochronic conduction to different target locations [56] . This presumably conveys time-sensitive information accurately and stably in time. On the other hand, a number of mechanisms are available to temporally vary axonal conduction and are listed in the Introduction section. To paraphrase, possibilities include variation in ion channel properties and ion concentrations, cellular morphology, the presence of subcellular organelles, and input from other axons or glia. Resolving which (and how) mechanisms contribute to the observed variations will be valuable but challenging. Local differences in velocities imply the existence of mechanisms acting locally, which may be observable optically. Combining the functional read-out of CMOS-based MEAs with super-resolution imaging of submicron diameter axons tagged with fluorescent molecular markers of, for example, ion channels or geometry may help to tease apart some relationships. However, much effort will be required to adapt existing set-ups for imaging cells on uneven and opaque surfaces of CMOS-based MEAs. The existence of candidate mechanisms, along with our previous observation of activity-dependent propagation plasticity [4] and the large variability observed in this study, hint that a neuron’s potential to temporally control its output may serve functions beyond isochronicity, including information processing in cortical circuits. Animal use All experimental protocols were approved by the Basel Stadt veterinary office according to Swiss federal laws on animal welfare. CMOS-based MEA Cortical networks were grown for many weeks over 11,011-electrode CMOS-based MEAs, which have enough spatial and temporal resolution to detect action potentials from any neuron lying on the array: 1.8 × 2.0 mm 2 area containing 8.2 × 5.8 μm 2 electrodes with 17.8 μm pitch (3,150 electrodes per mm 2 ), sampled at 20 kHz. The on-chip signal conditioning amplified (960X) and filtered (band-pass ~100–3.7 kHz) electrode voltage traces. The design choice to displace relatively large amplifiers to the outer side of the electrode array improved recorded signal quality by lowering circuit noise [28] . Owing to the array’s small feature sizes, a physical limit exists to the number of wires that can fit between electrodes. Therefore, an analogue switch matrix and 13,000 static random-access memory cells integrated underneath the electrode array sets the routing from the 126 read-out and/or stimulation channels to the desired electrodes. The electrode selection can be reconfigured within a few milliseconds to record in parallel from multiple neurons or selectively placed to sample an individual neuron at a subcellular resolution. Any electrode can supply a stimulus with an arbitrary waveform. For this paper, a positive-first biphasic voltage pulse, applied to one electrode at a time, was used in all experiments. Chips could survive months of culturing by passivating their surfaces with SiO 2 and Si 3 N 4 layers and by encapsulating bondwires in epoxy (Epo-Tek 302-3 M). Custom software on a personal computer, a field-programmable gate array and a microcontroller embedded in a custom circuit board were used to acquire and visualize data and control experiments. Unless otherwise noted, recorded spike waveforms were digitally band-pass filtered (200 Hz–3 kHz; see Supplementary Fig. S4 ). Signals were up-sampled up to 320 kHz following the Nyquist–Shannon sampling theorem and the Whitaker–Shannon interpolation formula to improve temporal measurements [57] . Matlab R2012a was used for data analysis. See refs 28 , 58 for circuit details. Platinum black deposition Depositing platinum black over electrodes reduces effective stimulation magnitude and artifact. Our protocol included applying a current of 180 μA simultaneously to all electrodes, using a platinum wire as a ground electrode immersed in the solution (0.7 mM hexachloroplatinic acid and 0.3 mM lead (II) acetate anhydrous). To improve deposition stability, an ultrasonic probe was inserted into the solution. Current was applied for 50–90 s. The first trial often produced a non-uniform deposition of platinum. Therefore, the chip was wiped with a cotton stick, and the procedure was repeated. Subsequent trials produced more uniform depositions, which appear black and can be optically verified under a microscope. Scanning configurations A first step in an experiment is to identify the locations of the neurons growing over the array, which was done by scanning a sequence of recording configurations across the array. A configuration is defined as how switches are set to connect a subset of the electrodes to the 126 read-out channels. A sequence consisted of either high-density blocks or random arrangements of recording electrodes. High-density blocks are advantageous for recording neurons’ footprints ( Fig. 1c ) within the same configuration. The largest possible contiguous block includes 6 × 17 electrodes requiring 108 configurations to access the whole array. However, neurons may not be detected if the network was silent when a given block was being recorded. As a somatic extracellular action potential can be detected across multiple electrodes (see Figs 1 and 4b ), scanning random configurations offers the advantage that a given neuron can be recorded in multiple configurations. Thus, for the same scanning time as used for block configurations, the chance of missing neurons during a silent period is reduced. Furthermore, to be confident that all active neurons were detected in a scan, configuration changes could be triggered by neural activity. We observed that some neurons would only fire during a network burst, and these thus served as suitable trigger sources. Scanning duration then depended on the activity level of the network. In Supplementary Fig. S1 , one such neuron was identified and used to ‘burst-trigger’ configuration changes after the occurrence of 10 network bursts ( Supplementary Fig. S1a ). Then, the spontaneous firing rates per electrode, throughout the whole duration of a configuration, were collected across the array ( Supplementary Fig. S1b ). In this manner, network topology could be non-invasively electrically ‘imaged’. Immunocytochemistry was done to verify the neural origin of the signals ( Fig. 1a , Supplementary Fig. S1c–d and Supplementary Movie 1 ). Although initial cell seeding was homogenous, neurons and glia migrated over days and weeks into more inhomogeneous arrangements. This necessitates rescanning on later dates to update neuron locations. Cell culture Techniques have been developed to maintain neural cultures and conduct experiments for many months [59] . Here, cells from embryonic day 18 Wistar rat cortices were dissociated in 2 ml of trypsin with 0.25% EDTA (Invitrogen) with trituration, and 10,000–40,000 cells were seeded over an area of ~12 mm 2 on top of the CMOS chip. A thin layer of poly(ethyleneimine) (Sigma), 0.05% by weight in borate buffer (Chemie Brunschwig) at 8.5 pH, followed by a 10-μl drop of 0.02 mg ml −1 laminin (Sigma) in Neurobasal (Invitrogen) were used for cell adhesion. After 24 h, the plating media was changed to growth media. Plating media consisted of 850 μl of Neurobasal supplemented with 10% horse serum (HyClone), 0.5 mM GlutaMAX (Invitrogen) and 2% B27 (Invitrogen). Growth media consisted of 850 μl of DMEM (Invitrogen) supplemented with 10% horse serum, 0.5 mM GlutaMAX and 1 mM sodium pyruvate (Invitrogen). Cultures matured for 3–4 weeks before experimentation, and experiments were conducted inside an incubator for a control of environmental conditions (36 °C and 5% CO 2 ). The MEAs were sealed using a Potter ring containing a hydrophobic membrane (fluorinated ethylene–propylene) that is selectively permeable to O 2 and CO 2 , and relatively impermeable to water vapour, bacteria and fungus [60] ; this allows long-term, non-invasive experimentation. To block synaptic activity, antagonists of fast synaptic receptors were used: 50 μM bicuculline methiodide, 100 μM 2-amino-5-phosphonovaleric acid and 10 μM 6-cyano-7-nitroquinoxaline-2, 3-dione (CNQX; Sigma), dissolved in growth media. These inhibit GABA-R, NMDA-R and AMPA-R, respectively, and effectively silence network activity. Cultures were allowed to equilibrate for an additional 30 min before experimentation. To visualize whole neurons, cells were sparsely transfected with a human synapsin I promoter driving DsRedExpress from the Callaway lab (Addgene plasmid 22909) using Lipofectamine 2000 (Invitrogen 11668) [35] . Images were collected at room temperature on a Leica DM6000 FS microscope with a × 10 long working distance objective lens and a Leica DFC 345 FX camera using the Leica Application Suite software. The monochrome camera captured 1600 × 1200 pixel images (0.35 μm per pixel edge) at a 12-bit resolution, which were later pseudo-coloured and inverted. Immunocytochemistry The neural source of extracellular signals was verified optically by immunocytochemistry. Cultures were fixed in 4% paraformaldehyde (Invitrogen) in phosphate-buffered saline (PBS) at pH 7.4 (PBS; Sigma) for 15 min at room temperature; washed twice with ice-cold PBS; permeabilized with 0.25% Triton X-100 (Sigma) in PBS for 10 min; and then washed in PBS three times for 5 min each time on a shaker. Next, unspecific binding of antibodies was blocked using PBS with 1% bovine serum albumin (BSA; Sigma) and 0.1% Tween 20 (Sigma) for 30 min. Then the primary antibody to MAP2 (Abcam ab5392) diluted to 1:500 in PBS with 1% BSA and 0.1% Tween 20 was added and left overnight at 4 °C on a shaker at low speed, and then washed three times in PBS for 5 min each time on the shaker. Next, the secondary antibody containing Alexa Fluor 647 (Invitrogen A21449) diluted to 1:200 in PBS with 1% BSA was added. After 1 h at room temperature in the dark, it was washed out three times with PBS for 5 min each time in the dark. Finally, to counterstain cell nuclei, 1 μg ml −1 4′,6-diamidino-2-phenylindole (Invitrogen D3571), dilution 1:1,000, was added for 1 min and washed twice with PBS. Coverslips were mounted with a drop of mounting medium (17970-25 CitiFluor AF1) and samples were stored in the dark at 4 °C. How to cite this article: Bakkum, D. J. et al . Tracking axonal action potential propagation on a high-density microelectrode array across hundreds of sites. Nat. Commun. 4:2181 doi: 10.1038/ncomms3181 (2013).